Imaging intraorganellar Ca2+at subcellular resolution using CEPIA The endoplasmic reticulum (ER) and mitochondria accumulate Ca 2+ within their lumens to regulate numerous cell functions. However, determining the dynamics of intraorganellar Ca 2+ has proven to be difficult. Here we describe a family of genetically encoded Ca 2+ indicators, named calcium-measuring organelle-entrapped protein indicators (CEPIA), which can be utilized for intraorganellar Ca 2+ imaging. CEPIA, which emit green, red or blue/green fluorescence, are engineered to bind Ca 2+ at intraorganellar Ca 2+ concentrations. They can be targeted to different organelles and may be used alongside other fluorescent molecular markers, expanding the range of cell functions that can be simultaneously analysed. The spatiotemporal resolution of CEPIA makes it possible to resolve Ca 2+ import into individual mitochondria while simultaneously measuring ER and cytosolic Ca 2+ . We have used these imaging capabilities to reveal differential Ca 2+ handling in individual mitochondria. CEPIA imaging is a useful new tool to further the understanding of organellar functions. The endoplasmic reticulum (ER) and mitochondria are membrane-bound intracellular organelles in eukaryotic cells that carry out vital functions. Both ER and mitochondrial membranes display Ca 2+ -transporting molecules whose function is to import Ca 2+ into the lumen against the concentration gradient. This uphill Ca 2+ transport is mediated in the ER membrane by sarco(endo)plasmic reticulum Ca 2+ ATPase (SERCA) [1] and in the inner mitochondrial membrane by the mitochondrial Ca 2+ uniporter (MCU) [2] . The organellar membranes also feature molecules that allow Ca 2+ to exit from the organelles to the cytosol: inositol 1,4,5-trisphosphate receptors and ryanodine receptors in the ER, and the Na + /Ca 2+ and H + /Ca 2+ exchangers in mitochondria [2] , [3] . Thus, the intraluminal Ca 2+ concentration in the organelles is tightly regulated, and may exceed that of cytosol by a large factor. Ca 2+ levels within the ER profoundly affect organelle function, and overload or depletion causes ER stress [4] . Within the mitochondrial matrix, Ca 2+ concentration regulates the rate of ATP production, and abnormal concentrations can lead to cell death or autophagic degradation of the mitochondria [2] . ER and mitochondrial structures are constantly being reorganized and close contacts form between the two types of organelles. These contact sites have recently been shown to be involved in diverse functions, including lipid biosynthesis, mitochondrial biogenesis and the transfer of Ca 2+ (refs 5 , 6 , 7 , 8 ). Both types of organelle are also involved in the regulation of cytosolic Ca 2+ concentrations. Release of Ca 2+ from the ER regulates contraction, fertilization, development, secretion and synaptic plasticity [3] . In addition, the ER luminal Ca 2+ concentration regulates Ca 2+ influx across the plasma membrane. Following a release of Ca 2+ from the ER, STIM1, which is present in the ER membrane, functions as a Ca 2+ transducer; it signals to the plasma membrane to activate the store-operated Ca 2+ entry mechanism (SOCE) [9] , [10] . SOCE is mediated by the molecular complex that includes Orai1, and is important for the activation of various cell functions, the best-studied example of which is the immune responses [9] . In contrast to the active role of the ER in Ca 2+ signalling, mitochondria have been considered to act as a passive Ca 2+ buffer [2] . However, recent results suggest that they may also have an active role as a source of Ca 2+ in the regulation of cytosolic Ca 2+ concentrations [11] . Although the importance of the ER and mitochondria as Ca 2+ -handling organelles is unequivocal, the mechanism by which organellar Ca 2+ concentrations regulate cellular processes remains elusive. New methods to dissect organellar Ca 2+ dynamics are expected to facilitate such studies. While small molecular Ca 2+ indicators cannot be precisely targeted to the organelles, limiting their use in living cells, genetically encoded Ca 2+ indicators (GECIs) can be targeted to organelles with the addition of appropriate tags [12] . Making use of this capability, GFP-based GECIs [13] , [14] , [15] , [16] , [17] , [18] , [19] , [20] , [21] , [22] , [23] and aequorin (a Ca 2+ -sensitive photoprotein) [24] have been used to measure intraorganellar Ca 2+ concentrations. FRET-type GFP-based GECIs were first used to measure intraluminal Ca 2+ concentration in the ER and were applied to different cell types [13] , [18] , [19] , [21] , [22] , [23] . This type of indicators uses wide visible wavelength bands for excitation and emission, often limiting the simultaneous use of other fluorescent molecules [25] , [26] . Subsequently, innovative modifications of the GFP molecule have yielded single-wavelength-excitation GECIs with various affinities to Ca 2+ for ER and mitochondrial Ca 2+ imaging [14] , [15] , [16] , [17] , [20] . Aequorin emits dim light, and simultaneous measurement with brighter fluorescence signals is not possible with most fluorescence microscopes. Although we have a wide variety of indicators, simultaneous Ca 2+ imaging of the ER and mitochondria has not been carried out, and improvement in the spatiotemporal resolution of organellar Ca 2+ is expected to enhance our understanding of intraorganellar Ca 2+ dynamics. For these reasons, and to study the functional interaction between the ER and mitochondria, a new type of GECIs with higher spatiotemporal resolution was required. This study reports on the generation of new organellar Ca 2+ indicators that allow simultaneous imaging of two subcellular compartments with high spatiotemporal resolution. They are optimized in terms of Ca 2+ affinity and dynamic range for organellar Ca 2+ imaging and come in colour variants for simultaneous measurement of multiple signals when they are used in appropriate combinations. Using them, intraorganellar Ca 2+ concentrations can be imaged at unprecedented spatiotemporal resolution. To illustrate the utility of the approach, we demonstrate high spatiotemporal resolution imaging of ER and mitochondrial Ca 2+ dynamics in living cells; we show the quantitative relationship between the ER Ca 2+ concentration and the extent of STIM1 puncta formation in the regulation of SOCE; and we show that inhomogeneity in mitochondrial Ca 2+ responses can be observed during apparently homogenous ER and cytosolic Ca 2+ changes, which suggest that there is a mechanism to regulate the influx of Ca 2+ into mitochondria. The new indicators described in this work will be valuable for further study of the roles of the ER and mitochondria, and of their functional interactions. 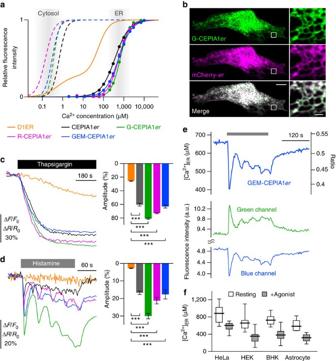Figure 1: Characterization of CEPIA. (a)In vitroCa2+titration curves of CEPIA1er(black solid), G-CEPIA1er(green solid), R-CEPIA1er(magenta solid), GEM-CEPIA1er(blue solid) compared with cfGCaMP2 (black dotted), G-GECO1.1 (green dotted), R-GECO1 (magenta dotted), GEM-GECO1 (blue dotted) and D1ER (orange). Fitted Hill plot curves are shown. Putative ranges of Ca2+concentration in the cytosol and ER are indicated (grey boxes). (b) Subcellular distribution of G-CEPIA1erand ER-targeted mCherry (with calreticulin signal sequence) in a HeLa cell. Note that the ER-signal sequence in G-CEPIA1eris different from that of mCherry-er. The images within the white boxes were expanded. Scale bars, 10 μm (left) and 1 μm (right). (c) Comparison of the responses of D1ER, CEPIA1er, G-CEPIA1er, R-CEPIA1erand GEM-CEPIA1erto thapsigargin (3 μM)-induced depletion of ER Ca2+in HeLa cells (n=12–31, mean±s.e.m.; ***P<0.001). Amplitude is defined as the extent of decrease in the fluorescence intensity or ratio after thapsigargin application normalized by the resting value. (d) ER Ca2+dynamics in response to histamine (10 μM) measured with D1ER, CEPIA1er, G-CEPIA1er, R-CEPIA1erand GEM-CEPIA1er(n=14–103, mean±s.e.m.; ***P<0.001). Amplitude is defined as the maximum decrease in ΔF/F0or ΔR/R0within a 30-s time window after histamine application. (e) Representative traces of the histamine-induced ER Ca2+dynamics visualized with GEM-CEPIA1erin a HeLa cell. Absolute [Ca2+]ER(upper) was estimated from the ratio of the blue to green (blue/green) fluorescence intensities (middle and bottom). (f) Cell type-specific variations of absolute [Ca2+]ERmeasured with GEM-CEPIA1er.Box plots for [Ca2+]ERin a variety of cell types before and after agonist stimulation (10 μM histamine for HeLa cells, 30 μM ATP for HEK cells and cultured astrocytes and 100 nM bradykinin for BHK cells;n=4–19) were shown. [Ca2+]ERafter agonist stimulation indicated the minimum value reached within 30 s after agonist application. The horizontal line within the box represents the median value, the upper and lower edges of the box represent 75 and 25% values and the whiskers represent the total range. Development of ER Ca 2+ indicator We began measuring ER Ca 2+ dynamics based on a lead variant of GCaMP2 (cfGCaMP2, see Methods), whereby fluorescence intensity increased 5.1-fold upon binding of Ca 2+ with a K d of 0.67 μM ( Supplementary Table 1 ). Since ER Ca 2+ concentration ([Ca 2+ ] ER ) is assumed to reach the sub-millimolar range, cfGCaMP2 was engineered to reduce its Ca 2+ binding affinity by a factor of ~1,000. We searched for low Ca 2+ affinity variants guided by extensive structure–function analyses based on site-directed mutagenesis in the calmodulin domain (See Methods). From among the 58 variants that were generated in our search we selected one with E31D/F92W/E104D/D133E substitutions that had a low Ca 2+ affinity ( K d =368 μM) and a large dynamic range ( F max / F min =4.2) ( Fig. 1a and Supplementary Fig. 1a,b ). After attaching ER localization and retention signal sequences, the low Ca 2+ affinity variant was expressed in HeLa cells. The engineered indicator protein colocalized with an ER marker [27] ( Supplementary Fig. 1c ). Upon addition of thapsigargin, an inhibitor of SERCA, a large reduction in fluorescence intensity was noted ( Fig. 1c ). Also, oscillatory fluorescence intensity decreased in response to histamine, which generates cytosolic Ca 2+ oscillations due to release of Ca 2+ from the ER via IP 3 Rs ( Fig. 1d ). Thus, the indicator successfully reports [Ca 2+ ] ER dynamics. We designated it C alcium-measuring organelle- E ntrapped P rotein I ndic A tor 1 in the ER (CEPIA1 er ). Figure 1: Characterization of CEPIA. ( a ) In vitro Ca 2+ titration curves of CEPIA1 er (black solid), G-CEPIA1 er (green solid), R-CEPIA1 er (magenta solid), GEM-CEPIA1 er (blue solid) compared with cfGCaMP2 (black dotted), G-GECO1.1 (green dotted), R-GECO1 (magenta dotted), GEM-GECO1 (blue dotted) and D1ER (orange). Fitted Hill plot curves are shown. Putative ranges of Ca 2+ concentration in the cytosol and ER are indicated (grey boxes). ( b ) Subcellular distribution of G-CEPIA1 er and ER-targeted mCherry (with calreticulin signal sequence) in a HeLa cell. Note that the ER-signal sequence in G-CEPIA1 er is different from that of mCherry- er . The images within the white boxes were expanded. Scale bars, 10 μm (left) and 1 μm (right). ( c ) Comparison of the responses of D1ER, CEPIA1 er , G-CEPIA1 er , R-CEPIA1 er and GEM-CEPIA1 er to thapsigargin (3 μM)-induced depletion of ER Ca 2+ in HeLa cells ( n =12–31, mean±s.e.m. ; *** P <0.001). Amplitude is defined as the extent of decrease in the fluorescence intensity or ratio after thapsigargin application normalized by the resting value. ( d ) ER Ca 2+ dynamics in response to histamine (10 μM) measured with D1ER, CEPIA1 er , G-CEPIA1 er , R-CEPIA1 er and GEM-CEPIA1 er ( n =14–103, mean±s.e.m. ; *** P <0.001). Amplitude is defined as the maximum decrease in Δ F / F 0 or Δ R / R 0 within a 30-s time window after histamine application. ( e ) Representative traces of the histamine-induced ER Ca 2+ dynamics visualized with GEM-CEPIA1 er in a HeLa cell. Absolute [Ca 2+ ] ER (upper) was estimated from the ratio of the blue to green (blue/green) fluorescence intensities (middle and bottom). ( f ) Cell type-specific variations of absolute [Ca 2+ ] ER measured with GEM-CEPIA1 er. Box plots for [Ca 2+ ] ER in a variety of cell types before and after agonist stimulation (10 μM histamine for HeLa cells, 30 μM ATP for HEK cells and cultured astrocytes and 100 nM bradykinin for BHK cells; n =4–19) were shown. [Ca 2+ ] ER after agonist stimulation indicated the minimum value reached within 30 s after agonist application. The horizontal line within the box represents the median value, the upper and lower edges of the box represent 75 and 25% values and the whiskers represent the total range. Full size image Multi-coloring of CEPIA We generated colour variants of CEPIA, based on recently developed cytosolic Ca 2+ indicators: R-GECO1 (red fluorescence), G-GECO1.1 (green fluorescence), and GEM-GECO1 (ratiometric blue/green fluorescence) [20] . After rigorous structure–function assessment (see Methods), we obtained R-CEPIA1 er ( K d =565 μM, F max / F min =8.8), G-CEPIA1 er ( K d =672 μM, F max / F min =4.7), and GEM-CEPIA1 er ( K d =558 μM, R max / R min =21.7; Fig. 1a and Supplementary Table 1 ). In vitro characteristics of these CEPIA variants, compared with those of original GECO, are summarized in Table 1 and Supplementary Fig. 2a–d . Table 1 Properties of CEPIA variants. Full size table We expressed the colour variants of CEPIA with ER-targeting signal sequences in HeLa cells. They localized to the ER [27] , [28] , and detected ER Ca 2+ oscillations with a high signal-to-noise ratio ( Fig. 1b–e and Supplementary Fig. 3a,b ). In HeLa cells, G-CEPIA1 er showed superior performance in signal amplitude over CEPIA1 er ( Fig. 1d ). To examine whether pH changes had any effect on the signal of CEPIA indicators ( Supplementary Fig. 2c ), we monitored pH dynamics in the ER using a pH sensor, enhanced yellow fluorescent protein (EYFP) [29] , [30] . There was no significant change in the fluorescence intensity of ER-localized EYFP ( Supplementary Fig. 4a–d ), verifying that the CEPIA responses are not due to pH changes in the ER. To measure the Ca 2+ affinity of CEPIA variants within the ER, we carried out Ca 2+ titration experiments in permeabilized HeLa cells. Stepwise changes in Ca 2+ concentration elicited dose-dependent fluorescence intensity changes in the presence of ionomycin to make the ER membrane permeable to Ca 2+ ( Supplementary Fig. 3c ). The K d values determined within the ER were almost equivalent to those measured in vitro ( Supplementary Fig. 3d ). Thus, we succeeded in expanding the hues of CEPIA variants. Estimation of [Ca 2+ ] ER Using ratiometric measurement of GEM-CEPIA1 er , we estimated [Ca 2+ ] ER in intact resting cells as varying between 620 and 860 μM in HeLa cells, HEK293A cells, BHK cells and cultured astrocytes; this decreased to 310–570 μM upon stimulation with agonists ( Fig. 1f ). The range of [Ca 2+ ] ER underlines the need to increase the indicator’s K d to >100 μM to provide faithful measurements of ER Ca 2+ dynamics, and explains the difficulty in imaging ER Ca 2+ dynamics using D1ER, which has a K d of ~60 μM (ref. 19 ; Fig. 1a,c,d ). Although CEPIA indicators had relatively high Hill coefficients ( n =1.4–2.0, Table 1 ), the relationship between Δ F / F max (or Δ R / R max ) and changes in [Ca 2+ ] is not highly distorted within the physiological [Ca 2+ ] ER range ( Supplementary Fig. 2e ). Subcellular ER Ca 2+ dynamics visualized with CEPIA We next examined whether CEPIA indicators are capable of detecting ER Ca 2+ dynamics at subcellular resolution. Agonists often induce Ca 2+ waves, which propagate throughout the cell after initiation in focal regions [31] , [32] . The wave is generated by the regenerative release of Ca 2+ from the ER, and it has been predicted that this mechanism creates an ‘inverse Ca 2+ wave’ within the ER. However, this prediction has not been tested using GECIs in live cells. We used G-CEPIA1 er imaging at a high frame rate (10–30 frames s –1 ) to visualize inverse Ca 2+ waves in the ER. Local decreases in [Ca 2+ ] ER were observed, initiating at the tips and propagating to the perinuclear region in HeLa cells ( Fig. 2a and Supplementary Movie 1 ). The time courses measured at two subcellular locations indicated a wave-like propagation of decreasing [Ca 2+ ] ER ( Fig. 2b,c ). The speed of these waves was 60.8±3.2 μm s –1 (mean±s.e.m. ), which matches cytosolic Ca 2+ waves with or without CEPIA expression ( Fig. 2d ). Similar observations were made with R-CEPIA1 er . Thus, CEPIA indicators have high spatiotemporal resolution. 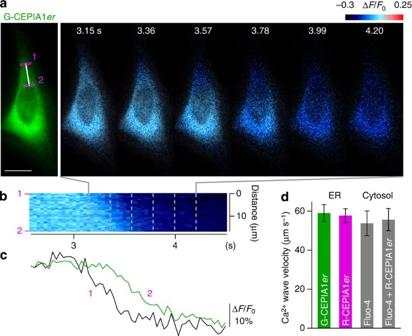Figure 2: Wave-like propagation of ER Ca2+release visualized with G-CEPIA1er. (a) Time-lapse images of wave-like decrease in the ER Ca2+concentration visualized with G-CEPIA1er. Perfusion of 10 μM histamine was started at 0 s. Scale bar, 20 μm. (b) Time course of ER Ca2+dynamics along the white line ina. (c) Comparison of ER Ca2+dynamics in two regions of interest ina. The fluorescence intensity was normalized by the initial intensity. Black line: region 1; green line: region 2. (d) The velocity of ER Ca2+wave measured with G-CEPIA1er(n=23, mean±s.e.m.) or R-CEPIA1er(n=20). For comparison, the velocity of cytosolic Ca2+wave measured with fluo-4 in cells without (n=8) or with R-CEPIA1erexpression (Fluo-4+R-CEPIA1er;n=6). There was no significant statistical difference among these values (P=0.93, one-way ANOVA). Figure 2: Wave-like propagation of ER Ca 2+ release visualized with G-CEPIA1 er . ( a ) Time-lapse images of wave-like decrease in the ER Ca 2+ concentration visualized with G-CEPIA1 er . Perfusion of 10 μM histamine was started at 0 s. Scale bar, 20 μm. ( b ) Time course of ER Ca 2+ dynamics along the white line in a . ( c ) Comparison of ER Ca 2+ dynamics in two regions of interest in a . The fluorescence intensity was normalized by the initial intensity. Black line: region 1; green line: region 2. ( d ) The velocity of ER Ca 2+ wave measured with G-CEPIA1 er ( n =23, mean±s.e.m.) or R-CEPIA1 er ( n =20). For comparison, the velocity of cytosolic Ca 2+ wave measured with fluo-4 in cells without ( n =8) or with R-CEPIA1 er expression (Fluo-4+R-CEPIA1 er ; n =6). There was no significant statistical difference among these values ( P =0.93, one-way ANOVA). Full size image We next examined whether CEPIA can be applied to intact tissue preparations. To do so, Ca 2+ dynamics were elucidated in the neuronal ER in response to synaptic inputs to Purkinje cell dendrites in cerebellar slice preparations. G-CEPIA1 er was expressed in Purkinje cells by Sindbis virus and was imaged with a two-photon microscope. G-CEPIA1 er expression was observed throughout the dendrites and into spines, matching the distribution of the ER in Purkinje cells ( Fig. 3a ). In response to parallel fibre stimulation, which induces Ca 2+ release from the ER by activating the metabotropic glutamate receptor [33] , we observed a long-lasting decrease in G-CEPIA1 er fluorescence intensity ( Fig. 3b and Supplementary Movie 2 ). The ER Ca 2+ dynamics could be visualized at the level of single spines ( Fig. 3c ). This response was not due to any pH change in the ER, because parallel fibre stimulation had no effect on pH within the ER measured by ER-targeted EYFP ( Supplementary Fig. 4e–g ) [29] , [30] . Thus, subcellular ER Ca 2+ imaging using CEPIA is applicable to tissue preparations that have retained three-dimensional structure, which often requires two-photon excitation. 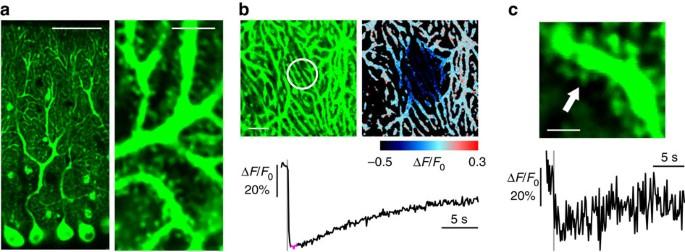Figure 3: Activity-dependent ER Ca2+dynamics in cerebellar Purkinje cells visualized with G-CEPIA1er. (a) G-CEPIA1er-expressing Purkinje cells in the cerebellar slice. Scale bars, 50 μm (left) and 5 μm (right). (b) PF-induced ER Ca2+dynamics in the dendrites of Purkinje cells. Time course of mean ΔF/F0within the white circle (indicated in the left image) indicates fluorescence decrease upon PF inputs (10 stimuli at 100 Hz, grey line). The pseudo-colour image that is the average of 10 consecutive frames (indicated as magenta in the time course of ΔF/F0) show local dynamics of luminal Ca2+. Scale bar, 10 μm. (c) PF-induced response in single spine of Purkinje cells. Representative time course of ΔF/F0within a spine indicated by the arrow. PF inputs (10 stimuli at 100 Hz, gray line) elicited ER Ca2+release within the spine. Scale bar, 2 μm. Figure 3: Activity-dependent ER Ca 2+ dynamics in cerebellar Purkinje cells visualized with G-CEPIA1 er . ( a ) G-CEPIA1 er -expressing Purkinje cells in the cerebellar slice. Scale bars, 50 μm (left) and 5 μm (right). ( b ) PF-induced ER Ca 2+ dynamics in the dendrites of Purkinje cells. Time course of mean Δ F / F 0 within the white circle (indicated in the left image) indicates fluorescence decrease upon PF inputs (10 stimuli at 100 Hz, grey line). The pseudo-colour image that is the average of 10 consecutive frames (indicated as magenta in the time course of Δ F / F 0 ) show local dynamics of luminal Ca 2+ . Scale bar, 10 μm. ( c ) PF-induced response in single spine of Purkinje cells. Representative time course of Δ F / F 0 within a spine indicated by the arrow. PF inputs (10 stimuli at 100 Hz, gray line) elicited ER Ca 2+ release within the spine. Scale bar, 2 μm. Full size image Simultaneous imaging of Ca 2+ dynamics in the ER and cytosol For simultaneous imaging of Ca 2+ dynamics in the ER and cytosol, we used the ratiometric small-molecule Ca 2+ indicator, fura-2 (excitation: 340–380 nm), together with G-CEPIA1 er or R-CEPIA1 er . ER Ca 2+ signals were a mirror image of the cytosolic Ca 2+ oscillations ( Supplementary Fig. 5a,b ). Although G-CEPIA1 er and R-CEPIA1 er are weakly excited at the excitation wavelengths of fura-2 ( Supplementary Figs 2a and 6a ), they had very little effect on the fura-2 fluorescence ratio ( Supplementary Fig. 6b ). Thus, it is possible to use G-CEPIA1 er and R-CEPIA1 er with fura-2. Either G-CEPIA1 er or GEM-CEPIA1 er can be co-expressed with R-GECO1 for simultaneous imaging of the ER and cytosolic Ca 2+ dynamics ( Supplementary Fig. 5c–f and Supplementary Movie 3 ). Reversal of the colours is also possible, and ER Ca 2+ imaging using R-CEPIA1 er can be simultaneously carried out with cytosolic Ca 2+ imaging using G-GECO1.1 or GEM-GECO1 ( Supplementary Fig. 5g,h ). Spectral bleed-through was minimal (<3%; Supplementary Fig. 6a ). These results show the versatility of CEPIA as an ER Ca 2+ indicator. Imaging of SOCE SOCE is a ubiquitous process to replenish ER Ca 2+ by inducing Ca 2+ influx from the extracellular space [10] , and has been shown to play an important role in the activation of immune cells [9] . SOCE has been previously analysed by measuring the increase in cytosolic Ca 2+ concentration ([Ca 2+ ] cyt ) after store depletion by SERCA inhibitors, such as thapsigargin and cyclopiazonic acid (CPA). However, it remains unclear whether SOCE induces an increase in [Ca 2+ ] cyt under physiological conditions [34] , [35] . Simultaneous Ca 2+ imaging in the ER and cytosol using G-CEPIA1 er and fura-2, respectively, provides a direct means to analyse Ca 2+ dynamics during SOCE. We found that stimulation of HeLa cells with histamine in the absence of extracellular Ca 2+ induced an increase in [Ca 2+ ] cyt and concomitant partial depletion of [Ca 2+ ] ER ( Fig. 4a , black lines). Removal of histamine resulted in a shift of [Ca 2+ ] cyt to [Ca 2+ ] ER in the continued absence of extracellular Ca 2+ . When Ca 2+ was reintroduced to the extracellular space (‘Ca 2+ add back’), a recovery of [Ca 2+ ] ER toward the pre-stimulation level was seen. During ER refilling with Ca 2+ , the increase in [Ca 2+ ] cyt was extremely small (Δ[Ca 2+ ] cyt =4.8±0.6 nM; Fig. 4c,d ) as compared with the large [Ca 2+ ] cyt increase (241±14 nM) observed after SERCA blockade by CPA or thapsigargin ( Fig. 4a and Supplementary Fig. 5i ). ER refilling was blocked by Gd 3+ , an Orai1 inhibitor [36] ( Fig. 4b ). When STIM1 was extrinsically expressed in HeLa cells, the [Ca 2+ ] cyt and ER Ca 2+ recovery rate during ‘Ca 2+ add back’ were significantly elevated ( Supplementary Fig. 5k,m ). These results indicate that, in HeLa cells, Ca 2+ influx via SOCE is rapidly taken up by SERCA without forming a high-amplitude cytosolic Ca 2+ signal unless STIM1 is overexpressed. We next examined Jurkat T cells stimulated with T-cell receptor activation. In these cells, although Ca 2+ influx via SOCE is partly taken up by SERCA as shown by the increase in [Ca 2+ ] ER , there was a significant increase in the cytoplasmic Ca 2+ concentration (Δ[Ca 2+ ] cyt =539±38 nM; Supplementary Fig. 5j ). Thus, unlike in HeLa cells, the rate of Ca 2+ influx via SOCE surpasses the ER Ca 2+ uptake rate in Jurkat T cells, and SOCE is capable of inducing an increase in [Ca 2+ ] cyt . 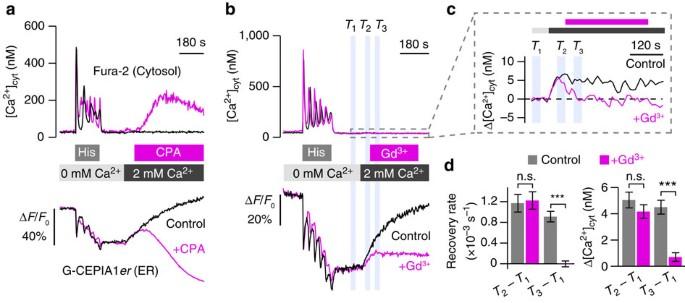Figure 4: Visualization of ER Ca2+dynamics during SOCE. (a,b) Ca2+dynamics in the ER (lower panels) and cytosol (upper panels) during SOCE. After histamine (10 μM)-induced Ca2+release in the absence of extracellular Ca2+, SOCE was induced by ‘Ca2+add back’, the reintroduction of Ca2+in the extracellular solution (black). To evaluate the contribution of SERCA-dependent Ca2+uptake by the ER, CPA was applied as indicated to the extracellular solution (a, magenta). The ER Ca2+refilling was inhibited by Gd3+(10 μM), an inhibitor of Orai1, during ‘Ca2+add back’ (b, magenta). (c) Magnified [Ca2+]cyttraces during ‘Ca2+add back’ in the upper panel ofb. (d) Changes in the ER Ca2+refilling rate and [Ca2+]cytin response to ‘Ca2+add back’ with or without Gd3+application. Left, the slope of linear fitting to the G-CEPIA1erfluorescence change during the intervalsT1toT3inb(lower panel) was obtained, and the indicated differences are shown. Right, the average [Ca2+]cytduring the intervalsT1toT3inb(upper panel) andcwas obtained, and the indicated differences are show.n=35 for control and 42 for Gd3+(mean±s.e.m.). ***P<0.001. Figure 4: Visualization of ER Ca 2+ dynamics during SOCE. ( a , b ) Ca 2+ dynamics in the ER (lower panels) and cytosol (upper panels) during SOCE. After histamine (10 μM)-induced Ca 2+ release in the absence of extracellular Ca 2+ , SOCE was induced by ‘Ca 2+ add back’, the reintroduction of Ca 2+ in the extracellular solution (black). To evaluate the contribution of SERCA-dependent Ca 2+ uptake by the ER, CPA was applied as indicated to the extracellular solution ( a , magenta). The ER Ca 2+ refilling was inhibited by Gd 3+ (10 μM), an inhibitor of Orai1, during ‘Ca 2+ add back’ ( b , magenta). ( c ) Magnified [Ca 2+ ] cyt traces during ‘Ca 2+ add back’ in the upper panel of b . ( d ) Changes in the ER Ca 2+ refilling rate and [Ca 2+ ] cyt in response to ‘Ca 2+ add back’ with or without Gd 3+ application. Left, the slope of linear fitting to the G-CEPIA1 er fluorescence change during the intervals T 1 to T 3 in b (lower panel) was obtained, and the indicated differences are shown. Right, the average [Ca 2+ ] cyt during the intervals T 1 to T 3 in b (upper panel) and c was obtained, and the indicated differences are show. n =35 for control and 42 for Gd 3+ (mean±s.e.m.). *** P <0.001. Full size image CEPIA imaging simultaneous with other fluorescent molecules Simultaneous time-lapse imaging of [Ca 2+ ] ER and other cellular processes should provide valuable information. We examined the possibility of simultaneously measuring [Ca 2+ ] ER and the subcellular distribution of STIM1, which senses the ER luminal Ca 2+ concentration and, upon ER Ca 2+ depletion, translocates to the subplasma membrane region to oligomerize [10] . Accumulating evidence suggests that the oligomerization of STIM1, which appears as a punctate structure of fluorescent protein-tagged STIM1, is a key determinant of SOCE [37] . We measured [Ca 2+ ] ER using GEM-CEPIA1 er and simultaneously imaged STIM1 dynamics using mCherry-STIM1 ( Fig. 5a,b and Supplementary Movie 4 ). Upon addition of histamine in the absence of extracellular Ca 2+ , [Ca 2+ ] ER began to decrease in an almost linear fashion. The formation of STIM1 puncta was considerably delayed, being observed only after [Ca 2+ ] ER fell below 600 μM. Thereafter, puncta formation proceeded alongside further decreases in [Ca 2+ ] ER . When Ca 2+ was added back to the extracellular solution after histamine washout, [Ca 2+ ] ER refilling began and the mCherry-STIM1 puncta decomposed. The relationship between [Ca 2+ ] ER and puncta formation could be fitted by Hill plot, with a Hill coefficient of 7.9 and a K 1/2 of 350 μM for puncta formation, and 9.7 and 530 μM for dissociation ( Fig. 5c ). Thus, the relationship between [Ca 2+ ] ER and puncta formation/dissociation exhibits considerable hysteresis. The difference of K 1/2 between puncta formation and dissociation was also observed using G-CEPIA1 er and mCherry-STIM1 ( Supplementary Fig. 5k,l ). These observations indicate that, as far as [Ca 2+ ] ER -dependent puncta formation of STIM1 is concerned, there is a threshold-like behaviour and suggest the existence of a mechanism that produces the delay in the dissociation of STIM1 puncta. Thus, CEPIA enables quantitative analysis of relationship between [Ca 2+ ] ER and STIM1 dynamics. 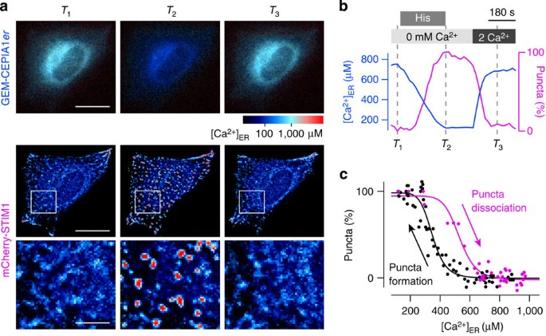Figure 5: Simultaneous imaging of STIM1 localization and ER Ca2+concentration. (a) The images of GEM-CEPIA1er(upper) and mCherry-STIM1 (middle) at three time points indicated inbas grey dotted lines (T1,T2andT3). The expanded images of mCherry-STIM1 within the white boxes were shown in the lower panels. Scale bars, 20 μm (upper and middle) and 5 μm (lower). (b) Time courses of ER Ca2+concentration (blue) and the number of mCherry-STIM1 puncta normalized with the minimum and maximum (magenta). As [Ca2+]ERwas depleted with histamine stimulation in the Ca2+-free solution, mCherry-STIM1 formed puncta (T2). After Ca2+addback in the external solution, [Ca2+]ERgradually recovered and mCherry-STIM1 puncta disappeared (T3). (c) The normalized number of mCherry-STIM1 puncta was plotted against ER Ca2+concentration during puncta formation (black) and dissociation (magenta). The plots obtained from three independent experiments were overlaid. The relationship between [Ca2+]ERand puncta formation can be fitted by Hill plot with a Hill coefficient of 7.9 and aK1/2of 350 μM for puncta formation, and 9.7 and 530 μM for puncta dissociation. Figure 5: Simultaneous imaging of STIM1 localization and ER Ca 2+ concentration. ( a ) The images of GEM-CEPIA1 er (upper) and mCherry-STIM1 (middle) at three time points indicated in b as grey dotted lines ( T 1 , T 2 and T 3 ). The expanded images of mCherry-STIM1 within the white boxes were shown in the lower panels. Scale bars, 20 μm (upper and middle) and 5 μm (lower). ( b ) Time courses of ER Ca 2+ concentration (blue) and the number of mCherry-STIM1 puncta normalized with the minimum and maximum (magenta). As [Ca 2+ ] ER was depleted with histamine stimulation in the Ca 2+ -free solution, mCherry-STIM1 formed puncta ( T 2 ). After Ca 2+ addback in the external solution, [Ca 2+ ] ER gradually recovered and mCherry-STIM1 puncta disappeared ( T 3 ). ( c ) The normalized number of mCherry-STIM1 puncta was plotted against ER Ca 2+ concentration during puncta formation (black) and dissociation (magenta). The plots obtained from three independent experiments were overlaid. The relationship between [Ca 2+ ] ER and puncta formation can be fitted by Hill plot with a Hill coefficient of 7.9 and a K 1/2 of 350 μM for puncta formation, and 9.7 and 530 μM for puncta dissociation. Full size image Intercellular heterogeneity of mitochondrial Ca 2+ signalling We examined whether CEPIA indicators can be utilized for Ca 2+ imaging in mitochondria. To cover the broad range of mitochondrial Ca 2+ concentrations (0.05–300 μM) [18] , [38] , [39] , three CEPIA variants with different Ca 2+ affinities were selected from the library: CEPIA2 ( K d =0.16 μM), CEPIA3 (11 μM) and CEPIA4 (59 μM; Fig. 6a , Supplementary Fig. 2f and Supplementary Table 1 ). These indicators were expressed in HeLa cells by adding the mitochondrial localization signal sequence [40] (CEPIA2 mt , CEPIA3 mt and CEPIA4 mt ) to their coding sequences. Expression colocalized with MitoTracker Red and was distinct from the ER ( Fig. 6b ). 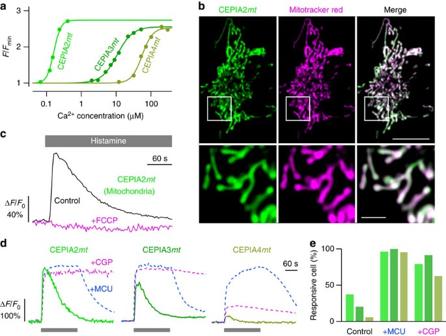Figure 6: Intercellular heterogeneity of mitochondrial Ca2+imaging visualized with CEPIA. (a) Ca2+titration curves of three mitochondria-targeted CEPIA variants (CEPIA2mt,Kd=160 nM,Fmax/Fmin=1.7; CEPIA3mt, 11 μM, 1.6; CEPIA4mt, 56 μM, 1.5). The measurements were performed at pH 8.0. (b) Representative images of HeLa cells expressing CEPIA2mt(left) co-stained with MitoTracker Red (middle). The merged images are shown in the right panels. The areas within the white boxes were expanded (lower). Scale bars, 10 μm (upper) and 2 μm (lower). (c) Time courses of mitochondrial Ca2+response using CEPIA2mtin HeLa cells prestimulated with FCCP (magenta) or DMSO (black). Representative trace of 11 cells for vehicle only (DMSO) and 15 cells for FCCP. (d) Representative traces of mitochondrial Ca2+dynamics upon stimulation with histamine (10 μM) in HeLa cells. To enhance mitochondrial Ca2+signal, rat MCU was extrinsically expressed (+MCU, blue) or the inhibitor of Na+/Ca2+exchanger CGP-37157 (10 μM) was applied (+CGP, magenta). (e) The percentage of cells with mitochondrial Ca2+responses upon histamine application measured with CEPIA2–4mtamong control HeLa cells, MCU-expressing cells (+MCU) and CGP-37157 (10 μM)-pretreated cells (+CGP). Figure 6: Intercellular heterogeneity of mitochondrial Ca 2+ imaging visualized with CEPIA. ( a ) Ca 2+ titration curves of three mitochondria-targeted CEPIA variants (CEPIA2 mt , K d =160 nM, F max / F min =1.7; CEPIA3 mt , 11 μM, 1.6; CEPIA4 mt , 56 μM, 1.5). The measurements were performed at pH 8.0. ( b ) Representative images of HeLa cells expressing CEPIA2 mt (left) co-stained with MitoTracker Red (middle). The merged images are shown in the right panels. The areas within the white boxes were expanded (lower). Scale bars, 10 μm (upper) and 2 μm (lower). ( c ) Time courses of mitochondrial Ca 2+ response using CEPIA2 mt in HeLa cells prestimulated with FCCP (magenta) or DMSO (black). Representative trace of 11 cells for vehicle only (DMSO) and 15 cells for FCCP. ( d ) Representative traces of mitochondrial Ca 2+ dynamics upon stimulation with histamine (10 μM) in HeLa cells. To enhance mitochondrial Ca 2+ signal, rat MCU was extrinsically expressed (+MCU, blue) or the inhibitor of Na + /Ca 2+ exchanger CGP-37157 (10 μM) was applied (+CGP, magenta). ( e ) The percentage of cells with mitochondrial Ca 2+ responses upon histamine application measured with CEPIA2–4 mt among control HeLa cells, MCU-expressing cells (+MCU) and CGP-37157 (10 μM)-pretreated cells (+CGP). Full size image Histamine application to mobilize ER Ca 2+ induced a rapid increase in mitochondrial Ca 2+ levels followed by a slow decay ( Fig. 6c ; black line). This mitochondrial Ca 2+ signal was abolished when the mitochondrial membrane potential was dissipated by carbonyl cyanide-p-trifluoromethoxyphenylhydrazone (FCCP) ( Fig. 6c ; magenta line). Only a subpopulation of cells showed a mitochondrial Ca 2+ response, and the fraction of responding cells decreased with the decreasing affinities of the CEPIA mt ( Fig. 6d,e and Supplementary Fig. 7a ). Enhancement of mitochondrial Ca 2+ , either by extrinsic expression of MCU or by suppression of Na + /Ca 2+ exchanger-mediated mitochondrial Ca 2+ clearance by CGP-37157, resulted in a striking increase in the fraction of cells displaying Ca 2+ signals. Under these conditions, sustained or oscillatory mitochondrial responses were observed in a large fraction of cells, and obvious saturation of CEPIA mt was observed in many cells ( Fig. 6d and Supplementary Fig. 7a ). We conclude that CEPIA mt successfully reports mitochondrial Ca 2+ signals, and that mitochondrial Ca 2+ dynamics during agonist stimulation have considerable cell-to-cell variation. Subcellular heterogeneity of mitochondrial Ca 2+ response In a fraction of cells, agonist stimulation elicited a mitochondrial Ca 2+ response throughout the cell. In the remaining cells, only a subpopulation of mitochondria responded with a Ca 2+ increase. For example, in the cell shown in Fig. 7a–c and Supplementary Movie 5 , mitochondrial Ca 2+ concentration ([Ca 2+ ] mt ) measured with CEPIA3 mt increased in region 2; the size of the increase is three times greater than that averaged over the entire cell. In contrast, there was no increase in [Ca 2+ ] mt in region 1. To exclude the possibility of regional variation in the CEPIA3 mt response, we applied a Ca 2+ ionophore, ionomycin. The same response was observed in both regions 1 and 2 ( Supplementary Fig. 7b,c ). Subcellular heterogeneity in mitochondrial Ca 2+ dynamics was also visualized by CEPIA2 mt ( Supplementary Fig. 7d–f ). These results indicate that there is a considerable subcellular variation in the capacity of mitochondria to take up Ca 2+ . 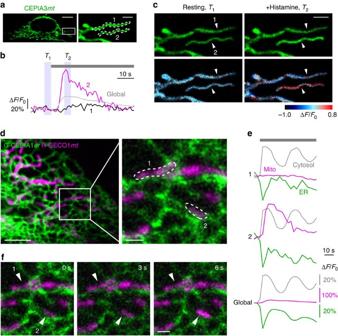Figure 7: Subcellular heterogeneity of mitochondrial Ca2+response. (a) Fluorescence image of a CEPIA3mt-expressing HeLa cell. The area within the white box was expanded. Scale bars, 10 μm (left) and 2 μm (right). (b) Time courses of mitochondrial Ca2+signal during 10 μM histamine application within the two regions of interest shown ina. Time course averaged over the entire cell was also shown (global). Averaged fluorescence images at resting state (T1, left blue box) and after histamine application (T2, right blue box) were indicated inc. (c) Upper, averaged fluorescence images at resting state (T1, left) and after histamine application (T2, right) as indicated inb. Lower, time-dependent changes in the fluorescence intensity were shown in pseudo-colour. Scale bar, 2 μm. (d) The fluorescence images of a HeLa cell expressing G-CEPIA1er(green) and mitochondria-localized R-GECO1 (R-GECO1mt, magenta). The area within the white box was expanded. Scale bars, 5 μm (left) and 1 μm (right). (e) Time courses of Ca2+signal in the mitochondria, ER and cytosol in a HeLa cell stimulated with 10 μM histamine within the two regions of interest indicated ind. Time courses averaged over the entire cell were also shown (Global). (f) The images of R-GECO1mt(magenta) and G-CEPIA1er(green) at three time points were shown. Representative images of six cells. Scale bar, 1 μm. Figure 7: Subcellular heterogeneity of mitochondrial Ca 2+ response. ( a ) Fluorescence image of a CEPIA3 mt -expressing HeLa cell. The area within the white box was expanded. Scale bars, 10 μm (left) and 2 μm (right). ( b ) Time courses of mitochondrial Ca 2+ signal during 10 μM histamine application within the two regions of interest shown in a . Time course averaged over the entire cell was also shown (global). Averaged fluorescence images at resting state ( T 1 , left blue box) and after histamine application ( T 2 , right blue box) were indicated in c . ( c ) Upper, averaged fluorescence images at resting state ( T 1 , left) and after histamine application ( T 2 , right) as indicated in b . Lower, time-dependent changes in the fluorescence intensity were shown in pseudo-colour. Scale bar, 2 μm. ( d ) The fluorescence images of a HeLa cell expressing G-CEPIA1 er (green) and mitochondria-localized R-GECO1 (R-GECO1 mt , magenta). The area within the white box was expanded. Scale bars, 5 μm (left) and 1 μm (right). ( e ) Time courses of Ca 2+ signal in the mitochondria, ER and cytosol in a HeLa cell stimulated with 10 μM histamine within the two regions of interest indicated in d . Time courses averaged over the entire cell were also shown (Global). ( f ) The images of R-GECO1 mt (magenta) and G-CEPIA1 er (green) at three time points were shown. Representative images of six cells. Scale bar, 1 μm. Full size image We tested a possible role for the ER in this inhomogeneous mitochondrial Ca 2+ response, since it has been postulated that ER Ca 2+ release is important for mitochondrial Ca 2+ responses [5] . To this end, simultaneous Ca 2+ imaging of the cytosol, ER and mitochondria was performed using GEM-GECO1, G-CEPIA1 er and R-GECO1 mt , respectively. Agonist stimulation induced a marked increase in [Ca 2+ ] mt in region 2 but not in adjacent mitochondria, including those in region 1. In contrast to the inhomogeneous mitochondrial response, [Ca 2+ ] ER and [Ca 2+ ] cyt showed similar responses in regions 1 and 2 ( Fig. 7d–f and Supplementary Movie 6 ). We also examined the subcellular heterogeneity in mitochondrial pH or membrane potentials (Ψ m ) as a potential mechanism of heterogeneous mitochondrial Ca 2+ responses [41] , [42] , [43] . Simultaneous measurement of [Ca 2+ ] mt and pH mt indicated that inhomogeneous Ca 2+ responses are not due to pH changes ( Supplementary Fig. 7g–j ). Neither did we find any heterogeneity in Ψ m , corresponding to mitochondrial Ca 2+ responses ( Supplementary Fig. 8 ). These results suggest that the inhomogeneous mitochondrial Ca 2+ response is generated by heterogeneity in the strength of ER-mitochondrial coupling or in the regulation of Ca 2+ uptake protein rather than in the amount of Ca 2+ released from the local ER or in pH or Ψ m . Ca 2+ concentrations within the ER and mitochondria control cytosolic Ca 2+ dynamics and regulate cell functions including ER stress and cell death [2] , [4] . Methods such as CEPIA that obtain direct information about intraorganellar Ca 2+ dynamics are therefore of great importance. The merits of CEPIA indicators for imaging ER or mitochondrial Ca 2+ concentrations can be summarized as follows. First, they have very high dynamic range and spatiotemporal resolution. This has allowed, for instance, the first imaging of an inverse Ca 2+ wave and synaptic activity-dependent ER Ca 2+ dynamics in neurons. Second, CEPIA allows simultaneous Ca 2+ imaging in the ER, mitochondria and cytosol with subcellular resolution. Third, CEPIA indicators are applicable to many cell types including intact neurons. Fourth, ratiometric measurement is possible with GEM-CEPIA1 er , whereby intraorganellar Ca 2+ concentrations can be determined independent of the indicator’s expression level. Fifth, the high signal-to-noise ratio and one-wave length measurement with G-CEPIA1 er and R-CEPIA1 er reduce the technical difficulty of organellar Ca 2+ imaging and obviate the requirement for a special imaging apparatus. Thus, CEPIA-mediated imaging methods should have broad utility in many cell biological studies. Indeed, work described in the paper addresses important cell functions. Influx of Ca 2+ from the extracellular space to the cytoplasm through SOCE is found in many types of cells [9] , [44] . The inhibition of SERCA (an ER Ca 2+ pump) by pharmacological means, such as thapsigargin and CPA, to deplete ER Ca 2+ has been the standard method to study the SOCE mechanism [9] . Now, using CEPIA, we have studied SOCE under physiological conditions, without SERCA inhibition. This revealed that [Ca 2+ ] cyt is held constant during SOCE activation in HeLa cells, although [Ca 2+ ] ER is sufficiently low to induce significant [Ca 2+ ] cyt increase when SERCA is inhibited. These results indicate that the balance between the SOCE and SERCA activities is important for the capacity of SOCE to induce sustained increase in [Ca 2+ ] cyt . In HeLa cells, SERCA activity is sufficiently high to take up Ca 2+ influx through SOCE. However, the balance can differ between cell types, and if it favors Ca 2+ influx there may be a large increase in [Ca 2+ ] cyt during SOCE activation. Indeed, we found that the balance favors Ca 2+ influx in Jurkat T cells, being consistent with the importance of SOCE in immune cells [9] . SOCE is a remarkable mechanism, in which [Ca 2+ ] ER regulates the Ca 2+ permeability in the plasma membrane. The ER Ca 2+ transducer of SOCE is STIM1, which senses [Ca 2+ ] ER and translocates to the subplasmalemmal ER domain to form punctate structures and recruits Orai1 for Ca 2+ influx through the plasma membrane. The steady-state [Ca 2+ ] ER dependence of the amplitude of ionic current carried by SOCE ( I CRAC ) and the subplasmalemmal translocation of STIM1 has been quantified [45] . I CRAC and STIM1 translocation were found to be nonlinear functions of [Ca 2+ ] ER with a Hill coefficient of ~4 and a K 1/2 of ~200 μM. This is consistent with the dissociation constant of the Ca 2+ -binding domain (EF-SAM) of STIM1 measured with a 45 Ca 2+ -binding assay ( K d =~250 μM) [46] . STIM1 deoligomerization for the termination of SOCE is thought to be mediated by ER Ca 2+ refilling [10] . Comparisons of the [Ca 2+ ] ER dependence of STIM1 puncta formation and dissociation have shown that K 1/2 of STIM1 puncta dissociation is lower than that of formation [47] , [48] . However, in these studies, STIM1 dynamics and [Ca 2+ ] ER had to be measured in separate cells, because both signals were measured using FRET between YFP and CFP. We found that extrinsic expression of STIM1 significantly increases both [Ca 2+ ] cyt and ER Ca 2+ refilling rate during SOCE. Thus, the comparison between cells with and without STIM1 expression requires caution. To circumvent this problem, we simultaneously measured STIM1 puncta formation/dissociation and [Ca 2+ ] ER in the same cells. Both STIM1 puncta formation and dissociation were highly nonlinear functions of [Ca 2+ ] ER . Furthermore, the K 1/2 of [Ca 2+ ] ER for puncta dissociation was greater than that for formation (530 and 350 μM for dissociation and formation, respectively). These results indicate that the STIM1 deoligomerization process is not a simple reversal reaction of STIM1 oligomerization. Within neurons the ER forms a continuous network throughout the cell (described as a ‘a neuron within a neuron’ that produces slowly propagating regenerative Ca 2+ signals using a conduction system based on IP 3 R and RyR [49] , [50] . However, neuronal ER Ca 2+ dynamics have previously been estimated only indirectly, by cytosolic Ca 2+ imaging. We have imaged Ca 2+ dynamics in the neuronal ER, in response to synaptic inputs to Purkinje cell dendrites in cerebellar slice preparations. Neuronal ER Ca 2+ dynamics are important for physiological functions such as synaptic plasticity [50] , but also for pathophysiological states including neurodegenerative diseases [4] , [51] . Thus, the application of CEPIA to intact neurons should provide a new imaging modality to analyse brain function. Accumulating evidence suggests that Ca 2+ dynamics in mitochondria are involved in the regulation of cell physiology and pathology, including autophagy, cell death, ATP synthesis, mitochondrial morphology and neurodegenerative diseases [2] , [8] . Mitochondria constantly undergo fusion and fission for the maintenance of functions [52] . Thus, subcellular inhomogeneity in mitochondrial functions is of great importance. Intracellular inhomogeneity in mitochondrial Ca 2+ dynamics was first proposed based on mitochondria-targeted aequorin measurements [53] , although these measurements did not have spatial resolution, and the inhomogeneity was inferred from the partial consumption of aequorin. Later, mitochondria-targeted GECIs were used to image the subcellular mitochondrial Ca 2+ response following agonist-induced ER Ca 2+ release [17] , [18] , [23] . These studies revealed that, after a rapid increase in [Ca 2+ ] mt in response to agonist stimulation, there is a considerable variation in the decay time course among the subpopulation of mitochondria within the cell, and a few minutes after the agonist stimulation only a minor subpopulation of mitochondria retained the increase in [Ca 2+ ] mt (refs 17 , 54 , 55 ). Our results showed that there is considerable intercellular and intracellular inhomogeneity in mitochondrial Ca 2+ responses after agonist-induced Ca 2+ release from the ER through IP 3 Rs, despite the fact that consistent cytosolic Ca 2+ increases were observed. These results are consistent with the observation using a small molecular Ca 2+ indicator [54] . Furthermore, simultaneous Ca 2+ imaging of the ER and mitochondria did not show any inhomogeneous ER Ca 2+ release. The inhomogeneity of the resting Ψ m also did not correlate with the inhomogeneity of Ca 2+ signal. These findings indicate that mitochondrial Ca 2+ responses involve more than simple, passive uptake of cytosolic Ca 2+ ; there must be a regulatory mechanism for Ca 2+ uptake. One possibility is that recently identified MCU [2] and its associate proteins such as mitochondrial calcium uptake 1 (MICU1) [55] , Mitochondrial Calcium Uniporter Regulator 1 (MCUR1) [56] , MCU regulatory subunit (MCUb) [57] and essential MCU regulator (EMRE) [58] as well as H + /Ca 2+ exchanger, Na + /Ca 2+ exchanger [2] are regulated in a subcellular region-specific manner. Another possibility is that ER–mitochondria tethering proteins such as mitofusin 2 (ref. 8 ) are inhomogeneously distributed, allowing region-specific transfer of Ca 2+ from the ER to mitochondria at the ER-mitochondrial junction [6] , [7] . Further study using CEPIA will provide clues to the mechanism coupling mitochondria and the ER. We created 58 variants of cfGCaMP2 and studied how their fluorescence intensity related to Ca 2+ levels. This work sheds light on the structure–function relationship of CaM-based indicators. Previous studies have reported that highly conserved glutamate residues at – Z position in each EF-hand motif are key determinants of the Ca 2+ sensitivity of CaM-based Ca 2+ indicators [11] , [13] , [59] . Here we further established that the substitution of glutamate with a non-acidic amino acid (E31A or E31Q) reduces not only the Ca 2+ binding affinity but also the dynamic range of the indicator. In contrast, conservative substitutions to aspartate reduced the Ca 2+ binding affinity, while maintaining the dynamic range. In line with this observation, a previous report showed that charge-reversing substitutions (E31K or E67K) resulted in a reduction of the dynamic range of cfGCaMP [59] . These results suggest that the acidic residue in – Z position is not only the key determinant of Ca 2+ binding affinity but is also important for the efficient conformational change upon Ca 2+ binding [60] . F92W and D133E substitutions that reduce Ca 2+ binding affinity without affecting the dynamic range have been previously reported for proteins possessing CaM-dependent enzymatic activity [61] . Combining these two types of substitutions synergistically reduced Ca 2+ binding affinity, which led to the generation of CEPIA indicators. This strategy may be applicable for the generation of ER and mitochondrial Ca 2+ indicators based on other CaM-based indicators. In summary, CEPIA-based imaging will contribute to the understanding of intraorganellar dynamics of Ca 2+ , and thus to elucidation of the functions of the ER and mitochondria in a variety of cells. Gene construction For creating a CEPIA library, we cloned cfGCaMP2 (GCaMP2 with amino-acid substitutions of M36L in CaM, and N105Y and E124V in circular permutated enhanced GFP (cpEGFP)) with ER retention signal sequence (SEKDEL) into a bacterial expression vector, pET19b (Novagen, USA), using primers 1 and 2 ( Supplementary Table 2 ). G-GECO1.1, R-GECO1 and GEM-GECO1 were also cloned into pET19b using primers 3 and 4. The CaM sequences in G-GECO1.1, R-GECO1 and GEM-GECO1 were swapped with that in cfGCaMP2 variants using primer 4–7. Site-directed mutagenesis was performed by PCR using primers 8–36. For mammalian expression of CEPIA variants in the ER and mitochondria, we cloned CEPIA into pCMV/myc/ER and pCMV/myc/mito vector (Invitrogen, USA) using primers 3, 4 and 37–39. For mitochondrial Ca 2+ imaging, we enhanced the specificity of mitochondrial localization by attaching the mitochondria targeting sequences in tandem [40] to CEPIA2–4 mt , R-GECO1 mt and GEM-GECO1 mt using primers 40–47. To enhance protein expression, GEM-CEPIA1 er was cloned into the CAG promoter-containing vector, pCIS, using primers 48 and 49. To express G-CEPIA1 er in the Purkinje cells, G-CEPIA1 er was cloned into pSinRep5 (Invitrogen) using primers 50–53. To localize EGFP and mCherry in the ER, EGFP and mCherry were cloned in the pcDNA3 D1ER [19] to attach calreticulin signal sequence using primers 54–59. To construct EYFP- er , EYFP was cloned from pcDNA3-YC4er [13] into pCMV/myc/ER vector using primers 60 and 61. To construct SypHer-dmito, we added an amino-acid substitution of C199S (ref. 62 ) in pHyper-dmito (Evrogen, Russia) using primers 62 and 63. To construct mCherry-STIM1, STIM1 was cloned from pApuro-GFP-STIM1 (ref. 63 ) into pShuttle2 vector using primers 60 and 64–66. Development of CEPIA indicators Ca 2+ affinity of cfGCaMP2 is primarily determined by calmodulin (CaM), which has four EF-hand motifs. We first tried the amino-acid substitutions that were used to reduce Ca 2+ affinity of the FRET-type ER Ca 2+ indicator, D1ER [19] , but the K d of cfGCaMP2 increased only to 14.5 μM ( Supplementary Fig. 1a , grey circle). Amino-acid substitutions at – Z position (12th amino-acid residue) of the EF-hand motifs were previously shown to reduce the Ca 2+ affinity of GFP-based Ca 2+ indicators [11] , [13] . When a non-acidic substitution (E31Q) at – Z in site I was introduced to cfGCaMP2, the K d increased to 64.9 μM. However, its dynamic range ( F max / F min ) was reduced to 2.5 ( Supplementary Fig. 1a , green circle). Another non-acidic substitution (E104Q) at – Z in site III produced no effect on the Ca 2+ affinity ( Supplementary Fig. 1a , light green circle). On the other hand, conservative E31D substitution in site I increased the K d to 14.5 μM without reducing the dynamic range. Therefore, we next systematically altered the glutamate residue at – Z positions (E31, E67, E104 and E140) to aspartate. The E67D variant had a K d of 9.2 μM, while E104D and E140D variants had 1.0 and 2.1 μM K d , respectively ( Supplementary Fig. 1a , cyan circles). We then examined whether combinations of multiple – Z substitutions would synergistically reduce the Ca 2+ affinity. The K d of E31D/E67D variant was strikingly increased to 470 μM, but its dynamic range was reduced to 2.6. Variants with other combinations of double substitutions had a K d of ~25 μM, and retained a high dynamic range. Combinations of three – Z substitutions, (E31D or E67D)/E104D/E140D, produced variants with a K d of ~130 μM ( Supplementary Fig. 1a , blue circles). Thus, we concluded that for further improvement of the indicator, we needed a different strategy. Previous reports have shown that a combination of F92W/D133E substitutions can inhibit Ca 2+ binding at site IV of CaM [61] . Based on these reports, we found that a cfGCaMP2 variant with F92W/D133E substitutions had a K d of 10.3 μM and a high dynamic range ( Supplementary Fig. 1a , orange circles). We next examined whether combinations of F92W/D133E and – Z substitutions synergistically reduce Ca 2+ affinity. Indeed, combinations of F92W/D133E and one of the – Z substitutions generated variants with a K d of 67–130 μM ( Supplementary Fig. 1a , magenta circles). We further combined the F92W/D133E substitutions with double – Z substitutions, (E31D or E67D) plus (E104D or E140D), and obtained variants with a K d of ~400 μM ( Supplementary Fig. 1a , magenta circles). Among them, a variant with E31D/F92W/E104D/D133E substitutions had a low Ca 2+ affinity ( K d =368 μM; Fig. 1a , solid black line) and a large dynamic range ( F max / F min =4.2; Supplementary Fig. 1a and Supplementary Table 1 ). To obtain the colour variants of CEPIA1 er , we first replaced the entire CaM domain of R-GECO1 with that of CEPIA1 er , and obtained a variant with a K d of 70.9 μM. Introduction of an additional – Z (E67D) substitution resulted in a variant with an optimal Ca 2+ affinity ( K d =565 μM) and a high dynamic range (8.8; Fig. 1a and Supplementary Table 1 ), which we designated R-CEPIA1 er . Using the same strategy, we replaced the CaM domain of G-GECO1.1 with CEPIA1 er CaM, and obtained a variant with a K d of 672 μM and a dynamic range of 4.7. This variant was designated as G-CEPIA1 er ( Fig. 1a and Supplementary Table 1 ). We next tried the same strategy in GEM-GECO1, but found that the dynamic range of the resulting indicator was markedly reduced ( R max / R min =1.1; Supplementary Table 1 ). As several amino-acid substitutions had been introduced to the CaM of GEM-GECO1 as compared with cfGCaMP2, we concluded that these additional substitutions are essential. Accordingly, we created a variant where we reintroduced the GEM-GECO1 substitutions while maintaining the E31D/F92W/E104D/D133E substitutions, creating a variant with a low Ca 2+ affinity and an increased dynamic range ( K d =225 μM, R max / R min =8.1; Supplementary Table 1 ). We further engineered the – Z positions, thus creating a variant with E31D/F92W/D133E/E140D substitutions with an optimal Ca 2+ affinity and a high dynamic range ( K d =558 μM, R max / R min =21.7; Fig. 1a and Supplementary Table 1 ). We designated this variant GEM-CEPIA1 er . Bacterial expression and in vitro spectroscopy BL21-CodonPlus(DE3)-RIL bacteria (Stratagene, USA) was transformed with the plasmids and incubated for 16–36 h at 37 °C in 2 × YT medium containing ampicillin and chloramphenicol (20 μg ml –1 ). The cells were resuspended in KCl/MOPS buffer (130 mM KCl, 50 mM MOPS, pH 7.2). After cell lysis with sonication, recombinant proteins were purified using TALON metal affinity resin (Clontech, USA) and dialyzed with Slide-A-Lyzer Dialysis Cassettes, 10 K MWCO (Thermo Fisher Scientific, USA). Ca 2+ and Mg 2+ titration curves of CEPIA variants were obtained by adding small aliquots of CaCl 2 or MgCl 2 to the recombinant indicators in a KCl/MOPS buffer containing 0 or 1 mM EGTA at pH 7.2. The Ca 2+ concentration carried over from the recombinant protein samples was estimated to be 2 μM. In the presence of 1 mM EGTA, the [Ca 2+ ] free at pH 7.2 was calculated as follows: where K d is the dissociation constant of CaEGTA (ref. 64 ). To estimate properties of CEPIA variants in mitochondria, titration experiments were performed in a KCl/HEPES buffer at pH 8.0 to mimic the mitochondrial environment [65] , containing 1 mM BAPTA, assuming a K d of 0.1 μM. Fluorescence intensity was measured with a spectrofluorometer (FP-750, Jasco, Japan) for each protein at excitation/emission wavelength; 488/512 nm for cfGCaMP2 and G-GECO1.1 variants, 562/584 nm for R-GECO1 variants and 395/460 nm and 395/510 nm for GEM-GECO1 variants. The obtained Ca 2+ -fluorescence intensity relationship was fitted by the following Hill plot equation using a least-square method in the Kaleidagraph software (Synergy Software, USA). For cfGCaMP2, G-GECO1.1 and R-GECO1 variants, For GEM-GECO1 variants, where R =( F at 460 nm)/( F at 510 nm). K d represents apparent dissociation constant, or the Ca 2+ concentration at which half of the indicator molecules bind to Ca 2+ . n represents Hill coefficient. The dynamic range of the indicator was calculated as the ratio of maximum and minimum fluorescence intensity or ratio ( F max / F min or R max / R min ). Fluorescence intensity at various Ca 2+ concentrations was standardized by the following equation: The absorbance spectra were measured with a spectrophotometer (DU-640 UV/VIS, Beckman, USA). To determine the molar extinction coefficient ( ε ), absorbance spectrum was measured first for each protein in KCl/MOPS buffer with or without 5 mM CaCl 2 . The extinction coefficient was calculated by dividing the peak absorbance by protein concentration. The protein concentration for G-CEPIA1 er , GEM-CEPIA1 er , G-GECO1.1 and GEM-GECO1 was calculated by measuring the absorbance following alkaline denaturation, assuming ε =44,000 M –1 cm –1 at 446 nm. For R-CEPIA1 er and R-GECO1, ε =38,000 M –1 cm –1 at 455 nm (ref. 20 ). Quantum yield (Φ) was calculated by using G-GECO1.1, R-GECO1 and GEM-GECO1 as a standard [20] . Animal experiments All animal experiments were carried out in accordance with the regulations and guidelines for Institutional Animal Care and Use Committee at The University of Tokyo and were approved by the institutional review committees of the Graduate School of Medicine, The University of Tokyo. Cell culture HeLa cells, HEK293A cells, BHK cells and astrocytes were cultured on collagen-coated dishes in DMEM supplemented with 10% foetal bovine serum, penicillin (100 U ml –1 ) and streptomycin (100 U ml –1 ). Jurkat T cells (E6-1) were maintained in RPMI medium (Gibco, USA) supplemented with 10% foetal bovine serum. An astrocytic culture with >95% purity was prepared by several replatings of the brain cell culture, which was obtained by 2.5% trypsin treatment and gentle trituration of the neocortices or the hippocampi of embryonic days 18–19 or postnatal days 1–3 Sprague–Dawley rat foetuses [66] . For Ca 2+ imaging, the cells were plated on collagen type-I-coated glass-bottom dishes (MatTek, USA) or Cell-Tak-coated dishes (Corning, USA) before imaging. Time-lapse Ca 2+ imaging Cultured cells were transfected using Lipofectamine 2000 (Invitrogen) 2 or 3 days before imaging. Jurkat T cells were electroporated using a MicroPorator (MP-100, Digital Bio) 1 day before imaging. For cytosolic Ca 2+ imaging using fura-2, cells were loaded with 5 μM fura-2 AM (Molecular Probes, USA) at room temperature (22–24 °C) for 40–60 min in 0.1% BSA-supplemented physiological salt solution (PSS) containing (in mM) 150 NaCl, 4 KCl, 2 CaCl 2 , 1 MgCl 2 , 5.6 glucose and 25 HEPES (pH 7.4). Before imaging, the loading solution was replaced with PSS without BSA. The images were captured using an inverted microscope (IX81, Olympus, Japan) equipped with a × 20 objective (numerical aperture (NA)=0.75, UPlanSApo, Olympus) or a × 40 objective (NA 0.90, UApo/340, Olympus), an electron-multiplying cooled-coupled device (EM-CCD) camera (ImagEM, Hamamatsu Photonics, Japan), a filter wheel (Lambda 10-3, Sutter Instrument, USA), a xenon lamp (ebx75) and a metal halide lamp (EL6000, Leica, Germany) at a rate of one frame per 2 or 3 s with the following excitation/emission filter settings: 472±15 nm/520±17.5 nm for G-GECO1.1, CEPIA1 er , G-CEPIA1 er , CEPIA2–4 mt and EYFP- er ; 562±20 nm/641±37.5 nm for R-GECO1, R-CEPIA1 er and mCherry-STIM1; 377±25 nm/466±20 nm and 377±25 nm/520±17.5 nm for GEM-GECO1 and GEM-CEPIA1 er ; 340±13 nm/510±42 nm and 365±6 nm/510±42 nm for fura-2; 440±10.5 nm/480±15 nm and 440±10.5 nm/535±13 nm for D1ER [19] , [20] . For analysis of the ratiometric indicators, we calculated the fluorescence ratio ( F 466 / F 520 for GEM-GECO1 and GEM-CEPIA1 er ; F 340 / F 365 for fura-2; F 535 / F 480 for D1ER). Photobleaching was corrected for using a linear fit to the fluorescence intensity change before agonist stimulation. All images were analysed with ImageJ software. To image subcellular ER Ca 2+ dynamics during agonist-induced Ca 2+ wave formation, we imaged HeLa cells expressing either G-CEPIA1 er or R-CEPIA1 er . Images were captured at a rate of one frame per 30–100 ms using a × 60 objective (NA 1.45, PlanApo TIRF, Olympus) and the metal halide lamp or an LED lamp (pE-100, CoolLED, UK). To evaluate Ca 2+ wave velocity in the ER and cytosol, images were normalized by the resting intensity, and a linear region of interest (ROI) was defined along the direction of wave propagation. A line-scan image was created by averaging 30 adjacent linear ROIs parallel to the original ROI, and time derivative was obtained to detect the time point that showed maximal change during the scan duration. Then, the time points were plotted against the pixel, and the wave velocity was estimated by the slope of the least-squares regression line. For mitochondrial Ca 2+ imaging with ER and cytosolic Ca 2+ , mitochondrial inner membrane potential or mitochondrial pH at subcellular resolution, we imaged HeLa cells with a confocal microscope (TCS SP8, Leica) equipped with a × 63 objective (NA 1.40, HC PL APO, Leica) at a rate of one frame per 2 or 3 s with the following excitation/emission spectra: R-GECO1 mt (552 nm/560–800nm), G-CEPIA1 er (488 nm/500–550 nm) and GEM-GECO1 (405 nm/500–550 nm); GEM-GECO1 mt (405 nm/500–550 nm), JC-1 (488 nm/500–550 nm and 488 nm/560–800nm); R-GECO1 mt (552 nm/560–800nm), SypHer-dmito (405 nm/500–550 nm and 488 nm/500–550 nm). For analysis of JC-1 and SypHer-dmito, we calculated the fluorescence ratio (488 nm/560–800 nm over 488 nm/500–550 nm for JC-1 (ref. 55 ); 488 nm/500–550 nm over 405 nm/500–550 nm for SypHer-dmito [62] ). To perform in situ Ca 2+ titration of CEPIA, we permeabilized the plasma membrane of HeLa cells with 150 μM β-escin (Nacalai Tesque, Japan) in a solution containing (in mM) 140 KCl, 10 NaCl, 1 MgCl 2 and 20 HEPES (pH 7.2). After 4 min treatment with β-escin, we applied various Ca 2+ concentrations in the presence of 3 μM ionomycin and 3 μM thapsigargin, and estimated the maximum and minimum fluorescent intensity ( R max and R min ), dynamic range ( R max / R min ), K d and n . For the estimation of [Ca 2+ ] ER based on the ratiometric measurement using GEM-CEPIA1 er ( Figs 1e,f and 5b and Supplementary Fig. 5f ), [Ca 2+ ] ER was obtained by the following equation: where R =( F at 466 nm)/( F at 510 nm), n =1.37 and K d =558 μM. To evaluate pH-dependent change of EYFP- er fluorescence ( Supplementary Fig. 4a–d ), we stimulated HeLa cells expressing EYFP- er in a PSS (adjusted to pH 6.8) containing monensin (10 μM, Wako) and nigericin (10 μM, Wako). Subsequently, the cells were alkalinized with a solution containing (in mM) 120 NaCl, 30 NH 4 Cl, 4 KCl, 2 CaCl 2 , 1 MgCl 2 , 5 HEPES and 5.6 Glucose (pH 7.4) [67] . Analysis of STIM1 dynamics STIM1 dynamics were analysed using the ImageJ software. To extract STIM1 puncta, the captured images were binarized after filtering (Gaussian Blur or Unsharp Mask). Then, particles greater than 2 pixels (corresponding to ~1.2 μm 2 ) were counted using the ‘Analyse Particles’ tool in ImageJ. The counts were normalized by the maximum values ( N puncta ) and plotted against the ER Ca 2+ levels (ER Ca 2+ ) ([Ca 2+ ] ER for GEM-CEPIA1 er and F / F 0 for G-CEPIA1 er ). Curve fitting was performed using the following Hill equation: where K 1/2 indicates the ER Ca 2+ level at half-maximal puncta formation and n represents Hill coefficient [68] . Imaging of subcellular localization of CEPIA All images were captured with a confocal microscope (TCS SP8) equipped with a × 63 objective at the following excitation/emission wavelengths: CEPIA1 er , G-CEPIA1 er , CEPIA2 mt , EGFP- er and EYFP- er (488 nm/500–550 nm), R-CEPIA1 er , mCherry- er and MitoTracker Red (Invitrogen; 552 nm/560–800nm) and GEM-CEPIA1 er (405 nm/420–550 nm). The obtained images were merged with ImageJ software. ER Ca 2+ imaging in cerebellar slices For Purkinje cell-specific expression of G-CEPIA1 er , we produced a Sindbis virus vector. The pSinRep5-G-CEPIA1 er vector was then used as the template for in vitro transcription using SP6 RNA polymerase (Ambion, USA). The RNA transcript and the helper RNA from DH(26S) cDNA template (Invitrogen) were cotransfected into BHK cells by electroporation. Twenty-four hours after transfection, the culture medium containing the infectious particles was harvested. Sindbis virus vector encoding EYFP- er was also produced with the same procedure. C57BL/6 mice (postnatal days 21–27) were deeply anaesthetized with pentobarbital, and the surface of cerebellar lobule 6 beside the midline was exposed by removing the cranium and dura. The tip of a glass pipette was backfilled with the viral solution. The glass pipette was then inserted into the cerebellum and 1 μl of viral solution was delivered at a rate of 200 nl min –1 using a micropump (Legato 130, KD Scientific, USA). Twenty-four hours after virus injection, parasagittal cerebellar slices (250 μm thickness) were prepared [69] . Mice were anaesthetized with diethyl ether and decapitated. The brain was removed and placed in ice-cold artificial cerebrospinal fluid (ACSF) bubbled with 95% O 2 /5% CO 2 . Slices were cut using a microslicer (PRO 7, Dosaka EM, Japan). The slices were incubated in a holding chamber containing ACSF bubbled with 95% O 2 and 5% CO 2 at 35 °C for 1 h and then returned to 23 °C. ACSF for slicing and incubation contained (in mM) 125 NaCl, 2.5 KCl, 2 CaCl 2 , 1 MgSO 4 , 1.25 NaH 2 PO 4 , 26 NaHCO 3 and 20 glucose. Slices were transferred to a recording chamber under a microscope, and continuously perfused with ACSF supplemented with 10 μM bicuculline (Tocris Bioscience, UK) and 10 μM NBQX (Tocris Bioscience) to block inhibitory postsynaptic potentials and accompanying Ca 2+ influxes. ACSF was bubbled with 95% O 2 and 5% CO 2 . Imaging was carried out with a two-photon microscope (TSC MP5, Leica) equipped with a water-immersion objective ( × 25, NA 0.95, HCS IR APO, Leica) and a Ti:sapphire laser (MaiTai DeepSee; Spectra Physics, USA). Excitation wavelength was 900–920 nm for both G-CEPIA1 er and EYFP- er . Data were acquired with time-lapse XY-scan mode (8 Hz) and analysed using ImageJ software. Fluorescence intensities were corrected for background fluorescence by measuring a non-fluorescent area. When necessary, photobleaching was corrected for using a linear fit to the fluorescence intensity change. For the focal stimulation of parallel fibres, square pulses (0.1 ms) were applied through stimulation pipettes (3–6 μm tip diameter) filled with ACSF. The stimulation intensity was adjusted within 4–5 V to induce G-CEPIA1 er signals with a range of ~20 μm in diameter. For EYFP- er , the stimulation intensity was fixed at 5 V. Experiments were carried out at room temperature. Statistics Two-tailed Student’s t -tests were performed to determine the significance if not stated otherwise. How to cite this article: Suzuki, J. et al . Imaging intraorganellar Ca 2+ at subcellular resolution using CEPIA. Nat. Commun. 5:4153 doi: 10.1038/ncomms5153 (2014).